Optimizing reaction paths for methanol synthesis from CO2hydrogenation via metal-ligand cooperativity As diversified reaction paths exist over practical catalysts towards CO 2 hydrogenation, it is highly desiderated to precisely control the reaction path for developing efficient catalysts. Herein, we report that the ensemble of Pt single atoms coordinated with oxygen atoms in MIL-101 (Pt 1 @MIL) induces distinct reaction path to improve selective hydrogenation of CO 2 into methanol. Pt 1 @MIL achieves the turnover frequency number of 117 h −1 in DMF under 32 bar at 150 °C, which is 5.6 times that of Pt n @MIL. Moreover, the selectivity for methanol is 90.3% over Pt 1 @MIL, much higher than that (13.3%) over Pt n @MIL with CO as the major product. According to mechanistic studies, CO 2 is hydrogenated into HCOO* as the intermediate for Pt 1 @MIL, whereas COOH* serves as the intermediate for Pt n @MIL. The unique reaction path over Pt 1 @MIL not only lowers the activation energy for the enhanced catalytic activity, but also contributes to the high selectivity for methanol. Hydrogenation of CO 2 into fuels and useful chemicals serves as an important process which helps to alleviate the dearth of fossil fuels [1] , [2] , [3] , [4] , [5] , [6] , [7] , [8] , [9] , [10] , [11] , [12] , [13] , [14] , [15] , [16] , [17] . According to both experimental and theoretical studies, CO 2 hydrogenation involves various reaction paths [4] , [5] , [6] . Even for the first step to activate CO 2 , CO 2 can be decomposed into CO*, transformed into carboxyl intermediate (COOH*), or hydrogenated into formate intermediate (HCOO*) [6] , [7] , [8] , [9] . Over practical catalysts, diversified reaction paths inevitably coexist, which induces the formation of different products such as CO, methane, formic acid, methanol, higher alcohols, and even gasoline, generally limiting the selectivity for the target product [10] , [11] , [12] , [13] , [14] . For instance, Cu/ZnO/Al 2 O 3 catalysts have already been applied to realize gas-phase CO 2 hydrogenation into methanol in industry, but suffer from the limited selectivity (<70%) for methanol and stringent reaction conditions (50–100 bar, 200–300 °C) [15] , [16] . Catalyzed by Cu/ZnO/Al 2 O 3 , CO 2 undergoes reverse water-gas shift path (RWGS) to produce CO* via the formation of COOH* species [17] . Since such catalysts also involve high energy barrier for the transformation of CO*, a large proportion of CO* is directly desorbed from the catalyst surfaces to form gaseous CO, competing over further hydrogenation into methanol [17] . Recently, constructing highly active interfaces such as Cu/CeO x , Cu/ZnO, and Cu/ZrO 2 interfaces has been reported to efficiently lower the energy barrier for the transformation of CO*, which not only increases the selectivity for methanol but also elevates the catalytic activity [18] , [19] , [20] , [21] , [22] , [23] . In addition, another pivotal approach is based on engineering the coordination environment of active metal atoms by alloying [24] , [25] . For instance, the fabrication of NiGa catalysts was found to suppress the RWGS path, thereby facilitating the production of methanol [26] . Co 4 N nanosheets were reconstructed into Co 4 NH x during aqueous CO 2 hydrogenation into methanol, wherein the amido-hydrogen atoms directly added CO 2 to form HCOO* [4] , . Despite of these achievements, it is still highly desiderated to efficiently control the reaction path for developing highly active and selective catalysts toward CO 2 hydrogenation. Herein, we demonstrate that metal-ligand cooperativity in Pt single atoms encapsulated in MIL-101 (Pt 1 @MIL) varies the reaction path and improves the selective hydrogenation of CO 2 into methanol relative to nanocrystal counterparts (Pt n @MIL). In Pt 1 @MIL, every Pt single atom and its coordinated O atoms compose an active center. During CO 2 hydrogenation, the turnover frequency (TOF) number of Pt 1 @MIL reaches 117 h −1 in DMF under 32 bar at 150 °C, being 5.6 times as high as that (21 h −1 ) of Pt n @MIL. Moreover, the selectivity for methanol reaches 90.3% over Pt 1 @MIL, whereas the major product for Pt n @MIL is CO with the selectivity of 57.5%. The cooperativity between Pt single atoms and their coordinated O atoms in Pt 1 @MIL enables the dissociation of H 2 to form O–H groups. The hydroxy H atoms add into CO 2 to produce HCOO* as the intermediates. As for Pt n @MIL, Pt–H is formed, wherein H atoms hydrogenate CO 2 into COOH* as the intermediates. The unique reaction path over Pt 1 @MIL not only lowers the activation energy for the enhanced catalytic activity, but also contributes to the high selectivity for methanol. Synthesis and structural characterizations of Pt 1 @MIL MIL-101 is a typical MOF which consists of μ 3 -oxo bridged Cr(III)-trimers cross linked by terephthalic acid [27] , [28] . The high specific surface area of S Langmuir = 5900 m 2 g −1 and large pore volume of ca. 2.0 cm 3 g −1 render MIL-101 high adsorption capacities, making it an attractive candidate for gas adsorption. As such, MIL-101 with an average particle size of 500 nm was synthesized based on previous literatures [27] , [28] (Supplementary Fig. 1 ), serving as the support in this work. In a typical synthesis of Pt 1 @MIL, K 2 PtCl 4 and NaBH 4 aqueous solutions were added into the flask containing MIL-101 aqueous solution via a syringe pump under magnetic stirring. In Pt 1 @MIL, the Pt mass loading was determined as 0.2% by inductively coupled plasma–atomic emission spectroscopy (ICP–AES). 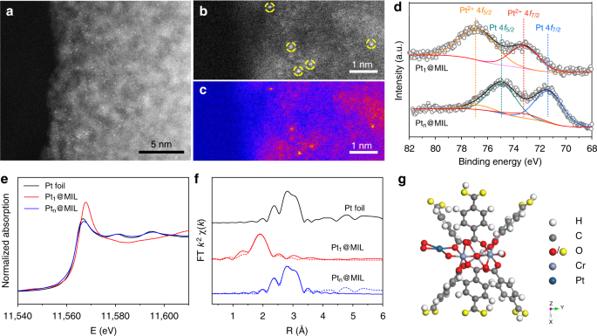Fig. 1 Structural characterizations of Pt@MIL.aHAADF-STEM image of Pt1@MIL.b,cMagnified HAADF-STEM image and its corresponding color-coded intensity map of Pt1@MIL. Pt single atoms marked in yellow circles were uniformly anchored in MIL-101.dXPS spectra of Pt 4ffor Pt1@MIL and Ptn@MIL.ePt L3-edge XANES profiles of Pt foil, Pt1@MIL, and Ptn@MIL.fPt L3-edge EXAFS spectra inRspace of Pt foil, Pt1@MIL, and Ptn@MIL. Pt foil was used as the reference.gStructural model of Pt1@MIL simulated by DFT calculations. Blue, violet, red, gray, and white spheres represent for Pt, Cr, O, C, and H atoms, respectively. The yellow spheres represent the oxygen atoms which are fixed at their positions in crystal Figure 1a shows a high-angle annular dark-field scanning transmission electron microscopy (HAADF–STEM) image of Pt 1 @MIL. As manifested by brightness, Pt atoms were atomically dispersed in MIL-101 in the absence of nanoparticles. To highlight the dopant atoms, the magnified HAADF–STEM image and its corresponding color-coded intensity map were shown in Fig. 1b, c , indicating the isolated distribution of Pt atoms. After Pt 1 @MIL was further washed for different rounds, the ratio of Pt to Cr remained almost unchanged, confirming that Pt single atoms were indeed anchored in MIL-101, rather than serving as a residual (Supplementary Fig. 2 ). By simply increasing the concentrations of K 2 PtCl 4 and NaBH 4 aqueous solutions, Pt n @MIL with the Pt mass loading of 1.0% was facilely synthesized. As shown in the HAADF–STEM image of Pt n @MIL, Pt nanocrystals with an average size of 1.8 nm were observed (Supplementary Fig. 3 ). The ratio of surface Pt atoms in Pt n @MIL was determined as 41.5% by CO pulse chemisorptions (Supplementary Fig. 4 ). To characterize the electronic properties of the obtained samples, we conducted X-ray photoelectron spectroscopy (XPS) measurements of Pt 1 @MIL and Pt n @MIL. As shown in Fig. 1d , the Pt species in Pt 1 @MIL was determined to be at Pt 2+ state. By comparison, most of Pt species in Pt n @MIL was at the metallic state, whereas a small portion of Pt was oxidized. Fig. 1 Structural characterizations of Pt@MIL. a HAADF-STEM image of Pt 1 @MIL. b , c Magnified HAADF-STEM image and its corresponding color-coded intensity map of Pt 1 @MIL. Pt single atoms marked in yellow circles were uniformly anchored in MIL-101. d XPS spectra of Pt 4 f for Pt 1 @MIL and Pt n @MIL. e Pt L 3 -edge XANES profiles of Pt foil, Pt 1 @MIL, and Pt n @MIL. f Pt L 3 -edge EXAFS spectra in R space of Pt foil, Pt 1 @MIL, and Pt n @MIL. Pt foil was used as the reference. g Structural model of Pt 1 @MIL simulated by DFT calculations. Blue, violet, red, gray, and white spheres represent for Pt, Cr, O, C, and H atoms, respectively. The yellow spheres represent the oxygen atoms which are fixed at their positions in crystal Full size image The X-ray absorption near-edge spectroscopy (XANES) and extended X-ray absorption fine structure (EXAFS) were measured to determine the electronic and coordination structures of Pt atoms in Pt@MIL catalysts. The Pt L 3 -edge XANES profiles in Fig. 1e indicate that the Pt species in Pt 1 @MIL were in a higher oxidation state than those in Pt n @MIL, according to the stronger intensity for white line. It is worth noting that the spectrum of Pt n @MIL was similar to that of Pt foil, indicating the metallic state of Pt species in Pt n @MIL, consistent with the XPS results (Fig. 1d ). As shown in EXAFS in R space (Fig. 1f ), Pt 1 @MIL exhibited a prominent peak at 2.01 Å from the Pt–O shell with a coordination number ( CN ) of 3.7 (Supplementary Table 1 ). No other typical peaks for Pt–Pt contribution at longer distances (>2.5 Å) were observed, revealing the isolated dispersion of Pt atoms throughout the whole Pt 1 @MIL. As for Pt n @MIL, a new peak at 2.76 Å was observed, corresponding to the Pt–Pt metallic bond with a CN of 7.4. To investigate the location and coordination of Pt single atoms in MIL-101, density functional theory (DFT) calculations were performed to establish the atomic model of Pt 1 @MIL. The building unit of MIL-101 comprises terephthalic linkers and an inorganic trimer. The trimer consists of three Cr atoms in an octahedral coordination. The vertices of octahedral coordination around each Cr atom are occupied by four O atoms from carboxylate groups in terephthalic linkers, one μ 3 O atom in the middle of Cr trimers, and one O atom from the terminal water or fluorine group. Both XPS and XANES results indicate an oxidation state assignment of Pt 2+ for Pt 1 @MIL (Fig. 1d, e ). In Pt 1 @MIL, the individual Pt atom was stabilized by O atoms in a planar four-coordinate geometry with one O atom in carboxyl, one dangling O connected with a Cr atom, and one O 2 moiety (Fig. 1g and Supplementary Fig. 5 ). This optimized model is consistent with the oxidation state of Pt 2+ indicated by XPS and XANES results, because Pt 2+ generally adopts the dsp 2 hybridization which results in the planar four-coordinate geometry. To further confirm the Pt oxidation states in this model, we have compared the charge of the Pt atom in Pt 1 @MIL with that in isolated Pt–O and O–Pt–O clusters as representatives of Pt 2+ and Pt 4+ (Supplementary Fig. 6 ). Based on Mullinken analysis, the charges of Pt atoms in Pt–O and O–Pt–O clusters are +0.72 and +1.52 e, respectively. The Pt single atom in Pt 1 @MIL is + 0.59 e charged, approximating to that in Pt–O cluster. Thus, the oxidation state of Pt in Pt 1 @MIL was assigned to +2. Moreover, the model of the Pt single atom coordinated with four O atoms in Pt 1 @MIL matches our EXAFS result in terms of the CN of Pt–O. Catalytic properties of Pt 1 @MIL for CO 2 hydrogenation The catalytic properties of the as-obtained Pt@MIL in CO 2 hydrogenation were evaluated in a slurry reactor with 10 mL of DMF under 32 bar of CO 2 /H 2 mixed gas (CO 2 :H 2 = 1:3) at 150 °C. As a benchmark, commercial Cu/ZnO/Al 2 O 3 (63 wt% Cu) was directly purchased from Alfa Aesar, with the ratio of surface Cu atoms to total atoms determined as 32.5% (Supplementary Fig. 7 ). For each catalytic test, the amounts of Pt 1 @MIL and Pt n @MIL were controlled at 500 and 240 mg, respectively, to keep the same amount (1.0 mg) of exposed Pt atoms, whereas 20 mg of Cu/ZnO/Al 2 O 3 was used. When the reaction was catalyzed by MIL-101, the product was below detection limit (Fig. 2a ). As for Pt 1 @MIL, 0.6 mmol of products were generated after 1 h, whereas the product yield was 0.12 mmol for Pt n @MIL. More importantly, the selectivity for methanol reached 90.3% over Pt 1 @MIL with the production of formic acid as the by-product (Fig. 2a ). With regard to Pt n @MIL, the major product was CO with the selectivity of 57.5%, while the selectivities for formic acid, methanol, and methane were 11.1%, 13.3%, and 18.1%, respectively (Fig. 2a ). In general, Pt-based heterogeneous catalysts have been reported to be selective to CO or methane during CO 2 hydrogenation [29] , [30] . In this case, Pt 1 @MIL did not give rise to the formation of gaseous products, behaving much differently from conventional Pt-based catalysts. As for Cu/ZnO/Al 2 O 3 , 0.16 mmol of methanol, 0.026 mmol of formic acid, and 0.024 mmol of CO were formed after 1 h (Fig. 2a and Supplementary Fig. 8 ). To compare the catalytic activity more accurately, we calculated the TOF numbers of these catalysts by only taking Pt atoms into account based on the reaction profile at the initial stage. The TOF number of Pt 1 @MIL reached 117 h −1 in DMF under 32 bar at 150 °C, being around 5.6 times that (21 h −1 ) of Pt n @MIL and 39 times that (3 h −1 ) of Cu/ZnO/Al 2 O 3 (Fig. 2b ). As a benchmark, the activity of Cu/ZnO/Al 2 O 3 in DMF solvent was comparable with the values obtained in a fixed-bed reactor [26] , [31] , [32] , [33] . We have further applied deuterated DMF (C 3 D 7 NO) as the solvent to replace DMF in CO 2 hydrogenation over Pt 1 @MIL under 32 bar at 150 °C. The TOF number of Pt 1 @MIL reached 107 h −1 in C 3 D 7 NO, almost equal to the corresponding values in DMF (Supplementary Fig. 9 ). Accordingly, the effect of proton transfer in DMF on CO 2 hydrogenation over Pt 1 @MIL could be neglected. Fig. 2 Catalytic performance of Pt@MIL in CO 2 hydrogenation. a Comparison of products obtained by using MIL-101, Pt 1 @MIL, Pt n @MIL, and commercial Cu/ZnO/Al 2 O 3 in DMF under CO 2 /H 2 mixed gas (CO 2 :H 2 = 1:3, 32 bar) at 150 °C after 1 h. b Comparison of TOF numbers of Pt 1 @MIL and Pt n @MIL in DMF under CO 2 /H 2 mixed gas (CO 2 :H 2 = 1:3, 32 bar) at different temperatures. c The Arrhenius plots of Pt 1 @MIL and Pt n @MIL. d Products obtained by conducting in-situ cycles over Pt 1 @MIL. For each cycle, the catalytic reaction proceeded under 32 bar of CO 2 /H 2 mixed gas (CO 2 /H 2 = 1:3) at 150 °C for 6 h. For each catalytic test, the amounts of Pt 1 @MIL and Pt n @MIL were controlled at 500 and 240 mg, respectively, to keep the same amount (1.0 mg) of exposed Pt atoms. Error bars represent standard deviation from three independent measurements Full size image To explore the differences in catalytic properties between Pt 1 @MIL and Pt n @MIL, we conducted a series of catalytic tests under 32 bar of CO 2 /H 2 mixed gas (CO 2 :H 2 = 1:3) at different temperatures. As shown in Fig. 2b , Pt 1 @MIL exhibited much higher catalytic activity than Pt n @MIL (Supplementary Figs. 10 and 11 ). Arrhenius plots were obtained based on the linear fitting of ln TOF vs. 1000/T (Fig. 2c ). The activation energy for Pt 1 @MIL was 76.4 kJ mol −1 , much lower than that (119.7 kJ mol −1 ) for Pt n @MIL. To investigate the size effect, Pt nanoparticles with an average size of 1.2 nm on MIL-101 were prepared and evaluated under 32 bar at 150 °C (Supplementary Fig. 12 ). The TOF number was calculated to be 22 h −1 which was lower than that (117 h −1 ) of Pt 1 @MIL and basically the same as that (21 h −1 ) of Pt n @MIL with 1.8-nm Pt nanoparticles (Supplementary Fig. 13 ). As such, Pt 1 @MIL exhibited higher catalytic activity and selectivity for methanol than Pt n @MIL even with tiny Pt clusters. To explore stability of Pt 1 @MIL, we performed successive rounds of reaction. For each round, the catalytic reaction proceeded at 150 °C for 1 h. After 10 rounds, the selectivity of methanol kept almost unchanged (Supplementary Fig. 14 ). Moreover, the HAADF-STEM image of the used Pt 1 @MIL (“used” refers to the catalyst after 10 rounds) showed that Pt atoms were still atomically dispersed in MIL-101 without the formation of nanoparticles (Supplementary Fig. 15 ). In addition, only 2.6% of Pt species in Pt 1 @MIL was leached after 10 rounds as revealed by ICP-AES. To further investigate the potential industrial application, we tested Pt 1 @MIL for successive in-situ cycles of reaction. For each cycle, the catalytic reaction proceeded under 32 bar of CO 2 /H 2 mixed gas (CO 2 /H 2 = 1:3) at 150 °C for 6 h without the removal of catalysts from the reactor during the whole test. After 16 in-situ cycles (96 h in total), Pt 1 @MIL led to the generation of about 14.6 mmol of methanol and 1.4 mmol of formic acid in total, exhibiting high long-term stability (Fig. 2d ). Accordingly, Pt 1 @MIL was highly stable during CO 2 hydrogenation, thereby exhibiting potential industrial application. Formation of hydroxyl groups in Pt 1 @MIL under H 2 We conducted DFT calculations to investigate the hydrogen dissociation on Pt 1 @MIL. 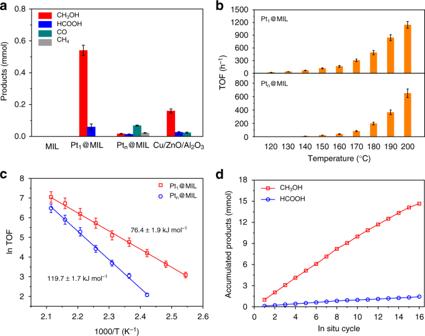Fig. 2 Catalytic performance of Pt@MIL in CO2hydrogenation.aComparison of products obtained by using MIL-101, Pt1@MIL, Ptn@MIL, and commercial Cu/ZnO/Al2O3in DMF under CO2/H2mixed gas (CO2:H2= 1:3, 32 bar) at 150 °C after 1 h.bComparison of TOF numbers of Pt1@MIL and Ptn@MIL in DMF under CO2/H2mixed gas (CO2:H2= 1:3, 32 bar) at different temperatures.cThe Arrhenius plots of Pt1@MIL and Ptn@MIL.dProducts obtained by conducting in-situ cycles over Pt1@MIL. For each cycle, the catalytic reaction proceeded under 32 bar of CO2/H2mixed gas (CO2/H2= 1:3) at 150 °C for 6 h. For each catalytic test, the amounts of Pt1@MIL and Ptn@MIL were controlled at 500 and 240 mg, respectively, to keep the same amount (1.0 mg) of exposed Pt atoms. Error bars represent standard deviation from three independent measurements Based on DFT calculations, the whole reaction path is divided into three elementary steps that include the dissociation of H 2 on Pt (step i), the formation of the first hydroxyl (step ii), and the formation of the second hydroxyl (step iii) (Supplementary Table 2 and Supplementary Fig. 16 ). Specially, H 2 is firstly dissociated on Pt to form Pt–H bonds. Afterwards, the two dissociated H atoms on Pt atoms stepwise migrates to the dangling O 2 moiety, resulting in the formation of two hydroxyl groups. Among these steps, step ii exhibits the highest energy barrier with the value of 0.79 eV, indicating that the formation of hydroxyl groups are able to proceed at 150 °C. To support this point, we carried out in-situ diffuse reflectance infrared Fourier transform spectroscopy (DRIFTS) measurements. 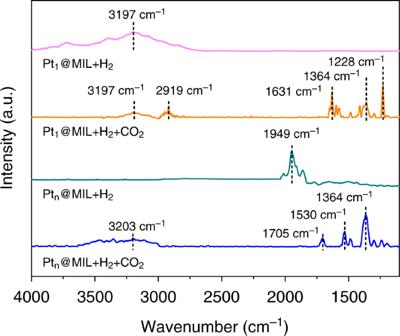Fig. 3 Adsorption properties of reactants on Pt@MIL. In-situ DRIFTS spectra of Pt1@MIL and Ptn@MIL after the treatment with H2, as well as H2and CO2in sequence at 150 °C Figure 3 shows the in-situ DRIFTS spectra of Pt 1 @MIL and Pt n @MIL after the treatment with H 2 at 150 °C for 0.5 h. As for Pt 1 @MIL, a peak at 3197 cm −1 appeared, corresponding to the stretching vibration of O–H. The observation of O–H and absence of Pt–H are consistent with the DFT results. With regard to Pt n @MIL, the peak at 1949 cm −1 was assigned to the stretching vibration of Pt–H. Therefore, Pt single atom activates its coordinated O atoms to adsorb the dissociated H atoms with the formation of two hydroxyl groups. As for Pt n @MIL, Pt nanoparticles directly dissociate H 2 to form Pt–H species. Fig. 3 Adsorption properties of reactants on Pt@MIL. In-situ DRIFTS spectra of Pt 1 @MIL and Pt n @MIL after the treatment with H 2 , as well as H 2 and CO 2 in sequence at 150 °C Full size image To investigate the role played by H atoms in hydroxyl groups, we have explored the kinetic isotope effect (KIE) with the use of D 2 in catalytic tests. When the reaction proceeded under CO 2 /D 2 mixed gas (CO 2 :D 2 = 1:3) at 150 °C, the TOF numbers of Pt 1 @MIL and Pt n @MIL were 21 h −1 and 13 h −1 , respectively (Supplementary Fig. 17a–b ). The KIE value refers to the ratio of the TOF using H 2 as the reactant gas to that using D 2 ( k H / k D ). As shown in Supplementary Fig. 17c , the KIE value of Pt 1 @MIL was 5.6 much higher than that (1.6) of Pt n @MIL. As such, the bond cleavage of O-D rather than Pt-D was involved in the reaction over Pt 1 @MIL. CO 2 hydrogenation paths The different adsorption properties of H atoms on Pt 1 @MIL and Pt n @MIL induced the variation of reaction paths in CO 2 hydrogenation. To investigate the reaction path, we calculated the addition of the first H atom into CO 2 . For Pt 1 @MIL, the energy of HCOO* is 0.26 eV lower than that of COOH* (Supplementary Fig. 18a–b and Tables 3 – 4 ). In this case, the first H atom adds to the C atom in CO 2 to form HCOO* as the stable intermediate on Pt 1 @MIL. In comparison, Pt n @MIL favors the generation of COOH* whose energy is 0.34 eV lower than that of HCOO* (Supplementary Fig. 18c–d and Tables 3 – 4 ). As such, the transformation of CO 2 into COOH* serves as the dominating reaction channel on Pt n @MIL. To support this point, we conducted in-situ DRIFTS measurements of Pt 1 @MIL and Pt n @MIL after the treatment with H 2 and CO 2 in sequence at 150 °C. For Pt 1 @MIL, the peak for O–H at 3197 cm −1 was still observed, but its intensity was weakened relative to the case when the sample was only treated with H 2 (Fig. 3 ). The peak at 1364 cm −1 was observed, indicating the formation of CO 2 δ- species [4] , [18] . Moreover, the peaks at 2919, 1631, and 1228 cm −1 also emerged, which were assigned to the stretching vibration of C–H, the asymmetrical and symmetrical stretching vibrations of the bidentate O–C–O in HCOO* species, respectively (Fig. 3 ). As for Pt n @MIL treated with H 2 and CO 2 in sequence relative to the one solely exposed to H 2 , the peak for Pt–H disappeared. Moreover, besides the peak for CO 2 δ- , the peaks at 3203, 1705, and 1530 cm −1 appeared, corresponding to the stretching vibration of O–H, the stretching vibration of C=O, and the bending vibration of C–O in COOH* species, respectively (Fig. 3 ). The in-situ DRIFTS results indicate that HCOO* and COOH* served as the intermediates for Pt 1 @MIL and Pt n @MIL, respectively, consistent with the theoretical results. The alteration of intermediates in CO 2 hydrogenation over Pt 1 @MIL and Pt n @MIL was further supported by quasi-situ XPS. Quasi-situ XPS measurements were conducted after the treatment of the samples with H 2 and CO 2 in sequence at 150 °C in a reaction cell attached to the XPS end-station. As shown in Fig. 4a , the C 1 s spectra exhibited four typical peaks at 284.6, 288.6, 289.5, and 291.0 eV, corresponding to benzene ring in MIL-101 (Ph), carboxyl group in MIL-101 (Ph-COO), HCOO*, and COOH*, respectively [18] , [34] , [35] , [36] . In addition, different species could also be distinguished in O 1 s spectra. Specifically, the peaks at 531.5 and 532.4 eV derived from the oxygen atoms in Ph–COO and HCOO*, respectively (Fig. 4b ). Two peaks at 530.0 and 531.1 eV were assigned to the carbonyl and hydroxyl species in COOH*, respectively (Fig. 4b ) [34] , [35] , [36] . As indicated by quasi-situ XPS spectra, HCOO* or COOH* was not observed for MIL-101. Therefore, the intermediates for Pt 1 @MIL and Pt n @MIL were determined as HCOO* and COOH*, respectively, consistent with in-situ DRIFTS results. Fig. 4 Mechanistic insight into remarkable activity of Pt 1 @MIL. a , b Quasi-situ XPS spectra of C 1 s and O 1 s for MIL-101, Pt 1 @MIL, and Pt n @MIL after the treatment with H 2 and CO 2 in sequence at 150 °C, respectively. c , d C and O K-edge XANES spectra for MIL-101, Pt 1 @MIL, and Pt n @MIL before/after the treatment with H 2 and CO 2 in sequence at 150 °C, respectively Full size image The intrinsic difference between HCOO* and COOH* lies in the exclusive existence of C–H bond in HCOO* and O–H bond in COOH*, which could be verified by C and O K-edge XANES measurements. 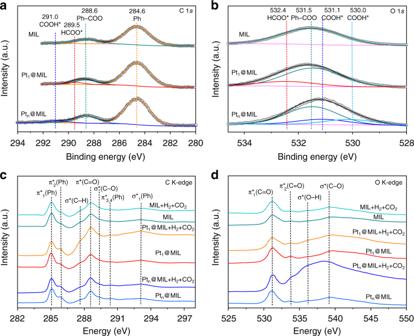Fig. 4 Mechanistic insight into remarkable activity of Pt1@MIL.a,bQuasi-situ XPS spectra of C 1sand O 1sfor MIL-101, Pt1@MIL, and Ptn@MIL after the treatment with H2and CO2in sequence at 150 °C, respectively.c,dC and O K-edge XANES spectra for MIL-101, Pt1@MIL, and Ptn@MIL before/after the treatment with H2and CO2in sequence at 150 °C, respectively Figure 4c shows the C K-edge XANES profiles of Pt 1 @MIL and Pt n @MIL before/after the treatment with H 2 and CO 2 in sequence at 150 °C. Before gas treatment, both Pt 1 @MIL and Pt n @MIL revealed the same XANES profiles which exhibited seven characteristic features. In detail, three features at 285.0, 285.9, and 290.3 eV were assigned to the excitations of the C=C π antibonding orbital for benzene ring in MIL-101 (π * (Ph)) [37] . Besides, the peaks at 287.6, 288.5, 289.4, and 293.1 eV corresponded to the excitations of the C–H antibonding orbital (σ * (C–H)), the C = O π antibonding orbital (π * (C=O)), the C–O antibonding orbital (σ * (C–O)), and the σ antibonding orbital for benzene ring in MIL-101 (σ * (Ph)), respectively [37] . After the treatment of MIL-101 with H 2 and CO 2 in sequence at 150 °C, the features were almost the same as the corresponding ones before the treatment. After the sequential gas treatment, the profiles of Pt 1 @MIL and Pt n @MIL both showed stronger feature of π * (C=O) relative to that without gas treatment, indicating the transformation of CO 2 . Moreover, the feature of σ * (C–H) became stronger for Pt 1 @MIL, but remained almost unchanged for Pt n @MIL. As such, only the species generated over Pt 1 @MIL contained C–H bond. As for O K-edge XANES, the features at 531.1 and 533.7 eV corresponded to the excitations of the π * (C=O), while the features at 536.1 and 539.1 eV were assigned to the O–H antibonding orbital (σ * (O–H)) and the C–O antibonding orbital (σ * (C–O)), respectively [38] (Fig. 4d ). After the exposure to H 2 and CO 2 in sequence at 150 °C, the feature of σ * (O–H) became significantly stronger for Pt n @MIL, but stayed almost the same for Pt 1 @MIL. Accordingly, only Pt n @MIL induced the generation of species containing O–H groups. In Pt 1 @MIL, every Pt single atom and its coordinated O atoms composed an active center. The metal-ligand cooperativity leads to the dissociation of H 2 to form hydroxyl groups, wherein hydroxy H atoms added into CO 2 to produce HCOO* as the intermediates. With regards to Pt n @MIL, Pt hydrides formed, offering H atoms to hydrogenate CO 2 into COOH* as the intermediates. In general, HCOO* is reported to be hydrogenated into HCOOH* and finally converted into methanol [6] , [9] . By comparison, besides forming HCOOH*, COOH* is also apt to lose the hydroxyl species to generate CO* species [6] , [18] . CO* can be either directly desorbed to form gaseous CO, or further hydrogenated into methane [6] . Thus, experiencing the reaction path via COOH* intermediate over Pt n @MIL leads to the formation of gaseous products. In conclusion, the metal-ligand cooperativity in Pt 1 @MIL was found to induce distinct reaction path and improve selective hydrogenation of CO 2 into methanol relative to Pt n @MIL. According to mechanistic studies, CO 2 was hydrogenated into HCOO* as the intermediate for Pt 1 @MIL, whereas COOH* served as the intermediate for Pt n @MIL. The unique reaction path over Pt 1 @MIL both lowered the activation energy for the enhanced activity and led to the high selectivity for methanol. Upgrading the catalysts from nanocrystals to single atoms not only enhances the atomic utilization efficiency, but also alters the catalytic mechanisms such as the adsorption of reactants or intermediates on catalysts and the reaction path. This strategy offers a powerful means to improve the catalytic performance for CO 2 hydrogenation, and extends our understanding of single-atom catalysis. Synthesis of MIL-101 The synthesis of MIL-101 followed a reported method [28] . Specifically, 2 g of Cr(NO 3 ) 3 ·9H 2 O, 830 mg of terephthalic acid, and 0.225 mL of HF aqueous solution (40.0% in mass fraction) were added into 25 mL of water in a 50-mL beaker, followed by stirring at room temperature for 15 min. Then, the solution was transferred into a 50-mL Teflon-lined autoclave and heated at 220 °C for 8 h. After the solution was cooled to room temperature, the product was collected by centrifugation, washed three times with water. For further purification, the solid product was sequentially stirred in 200 mL of ethanol solution (95% ethanol with 5% H 2 O) at 80 °C for 24 h, 300 mL of NH 4 F aqueous solution (30 mM) at 70 °C for 24 h, and 200 mL of water at 90 °C for 3 h. The product was collected by centrifugation, and then dried at 60 °C under vacuum. Synthesis of Pt@MIL In a typical synthesis of Pt 1 @MIL, 100 mg of MIL-101 were dispersed in 60 mL of water in a 250-mL flask under magnetic stirring for 10 min. 10.1 mL of K 2 PtCl 4 aqueous solution (0.1 mM) and 10.1 mL of NaBH 4 aqueous solution (0.1 mM) were added into the flask through a two-channel syringe pump at a rate of 2 mL h −1 under magnetic stirring at room temperature. The sample was washed three times with water, and dried at 60 °C under vacuum. Further ICP result determined that the mass loading of Pt was 0.2%. The synthetic procedure for Pt n @MIL with the Pt loadings of 1.0% was similar to that for Pt 1 @MIL, except for increasing the amounts of K 2 PtCl 4 and NaBH 4 . For Pt n @MIL, 10.4 mL of K 2 PtCl 4 aqueous solution (0.5 mM) and 10.4 mL of NaBH 4 aqueous solution (0.5 mM) were added into the flask through a two-channel syringe pump at a rate of 10 mL h −1 under magnetic stirring at room temperature. The synthesis of Pt nanoparticles with an average size of 1.2 nm was similar to that of Pt n @MIL except for the concentration of precursors. Specially, 100 mg of MIL-101 were dispersed in 60 mL of water in a 250-mL flask under magnetic stirring for 10 min. 10.4 mL of K 2 PtCl 4 aqueous solution (0.3 mM) and 10.1 mL of NaBH 4 aqueous solution (0.5 mM) were added into the flask through a two-channel syringe pump at a rate of 10 mL h −1 under magnetic stirring at room temperature. XAFS measurements The XAFS measurements were carried out at Pt L 3 -edge (11564 eV) on the BL14W1 beamline [39] of Shanghai Synchrotron Radiation Facility. The XAFS data of Pt@MIL were recorded in fluorescence mode by using a Ge solid-state detector. The calibration of the energy was based on the absorption edge of pure Pt foil. The data extraction and fitting were carried out by using Athena and Artemis codes. As for XANES, the normalized absorption refers to the experimental absorption coefficients vs. energies μ ( E ) after background subtraction and normalization procedures. As for EXAFS, the first-shell approximation was adopted to analyze the Fourier transformed data in R space of the Pt–O shell, while metallic Pt model was used to analyze that of the Pt–Pt shell. To determine the passive electron factors ( S 0 2 ), the experimental Pt foil data were fitted while the CN of Pt–Pt was fixed as 12. Afterwards, S 0 2 was fixed for further analysis. The parameters such as bond distance ( R ), CN , and Debye Waller ( D.W .) factor around the absorbed atoms were variable during the fitting process. DFT calculations Density functional theory (DFT) calculations were performed using Gaussian program [40] to explain the interaction mechanism between CO 2 and Pt 1 @MIL, a cluster with 30 O atoms, 48 C atoms, 3 Cr atoms, 32 H atoms, and 1 Pt atom was adopted to simulate Pt 1 @MIL. The six carboxylate terminals on the top of benzene ring were saturated by hydrogen atoms (COO − → COOH) and the twelve oxygen atoms were fixed at their crystal positions during geometric optimization. We made calculations with B3LYP-D3 functional [41] implemented in Gaussian with the combination of the Grimme’s third generation dispersion correction (D3) [42] . For structural optimization, the standard Gaussian-type basis sets 6–31 G(d) [43] was used for C, O, and H atoms and LANL2DZ [44] sets for metal atoms. As for the calculation of reaction paths, we used the optimized structure for a higher-precision single-point energy calculation. In the level, the basis sets for describing C, O, and H atoms was replaced by 6–311++G(d, p) [45] , whereas the basis sets for metal atoms still adopted LANL2DZ. In order to simulate the periodic Pt (111), we used Vienna ab initio simulation package (VASP) [46] , [47] . The projector augmented wave (PAW) method was used to describe the interaction between ions and electrons [48] . The nonlocal exchange correlation energy was evaluated using the Perdew–Burke–Ernzerhof functional [49] . A plane wave basis set with a cutoff energy of 400 eV and a 1 × 1 × 1 k -point grid generated by the Monkhorst–Pack method were used to describe the Brillouin zone for geometric optimization. The atomic structures were relaxed using either the conjugate gradient algorithm or the quasi-Newton scheme as implemented in the VASP code until the forces on all unconstrained atoms were ≤0.02 eV Å −1 . Catalytic tests of Pt@MIL catalysts in CO 2 hydrogenation The hydrogenation of CO 2 was conducted in a 100-mL slurry reactor (Parr Instrument Company). In a typical catalytic test, the reactor was charged and discharged with 32 bar of mixed gas (CO 2 :H 2 = 1:3) at room temperature for three times, after the addition of 10 mL of DMF and certain amounts of catalysts into the Teflon inlet. For a catalytic test, the weights of Pt 1 @MIL and Pt n @MIL were controlled at 500 and 240 mg, respectively, so as to keep the same amount (1.0 mg) of exposed Pt in each catalyst. The reaction proceeded under stirring with a rate of 300 rpm and 32 bar of mixed gas (CO 2 :H 2 = 1:3) at 150 °C. After the completion of the reaction, the gaseous products were determined by GC-FID and GC-TCD. The reaction mixture in liquid phase was collected by centrifugation at 11,180 × g for 2 min. The test solution contained 50 μL of chloroform, as an internal standard, and 1 mL of the reaction mixture. 100 μL of the test solution was dissolved in 0.4 mL of DMSO-d 6 for the measurements of 1 H NMR. For each data point, the catalytic tests were repeated thrice. For the stability of Pt 1 @MIL, we applied two methods including successive reaction rounds and in-situ cycles. The addition of catalysts, solution, and reaction gases followed the same procedure as a typical catalytic test. Successive reaction rounds were carried out with the collection of catalysts for each round. Specially, after the proceeding of reaction at 150 °C for 1 h, both gaseous and liquid products were detected. Meanwhile, the catalysts were collected via centrifugation and washed thrice with DMF, followed by being re-added to the slurry reactor for the next round. In-situ cycles were carried out without opening the slurry reactor to collect the catalysts. For each cycle, after the proceeding of reaction at 150 °C for 6 h, both gaseous and liquid products were taken through tubes for detection. The TOF was calculated based on the equations. TOF = n_CO2/( t × n_surface Pt atoms) = n_CO2×μ _Pt/( t × m_surface Pt atoms)
 (1) 
    m_surface Pt = m_cat× w × r_surface
 (2) In this equation, n CO2 represents the mole of converted CO 2 molecules. t is the reaction time. n surface Pt atoms represents the mole of surface Pt atoms. μ Pt is the weight of one mole of Pt atoms. m surface is the weight of surface Pt species in the catalysts. m cat is the weight of catalysts. w represents the mass loading of Pt species. r surface represents the ratio of surface Pt atoms to total Pt atoms. For Pt 1 @MIL, we assumed that all the Pt atoms were exposed on the surface, so that r surface is 100.0%. For Pt n @MIL, r surface was determined as 41.5% via CO pulse chemisorptions In-situ DRIFTS tests The instrument for in-situ DRIFTS experiments was composed of an elevated-pressure cell (DiffusIR Accessory PN 041-10XX) and a Fourier transform infrared spectrometer (TENSOR II Sample Compartment RT-DLaTGS). The resolution of wavenumber was 4 cm −1 at 150 °C. The background spectrum was obtained after a N 2 flow (1 bar) for 0.5 h at 150 °C. Then, 1 bar of H 2 was allowed to flow into the cell at the rate of 30 sccm at 150 °C for 0.5 h, followed by flowing with 1 bar of N 2 at the rate of 30 sccm at 150 °C for 0.5 h. To detect the species generated after the treatment of the samples with H 2 and CO 2 in sequence, 1 bar of H 2 was allowed to flow into the cell at the rate of 30 sccm at 150 °C for 0.5 h, followed by flowing with 1 bar of N 2 at the rate of 30 sccm at 150 °C for 0.5 h. Then, 1 bar of CO 2 was allowed to flow into the cell at 25 °C for 30 min, followed by purging with 1 bar of N 2 at 25 °C for 30 min. Quasi-situ XPS measurements Quasi-situ XPS measurements were performed at the photoemission end-station on the BL10B beamline of National Synchrotron Radiation Laboratory (NSRL, China). The samples were exposed to 1 bar of H 2 and CO 2 in sequence at 150 °C for 0.5 h. Afterwards, the samples were moved to the analysis chamber for further XPS analysis. Instrumentations TEM, HAADF–STEM, and STEM–EDX images were collected on a JEOL ARM-200F field-emission transmission electron microscope operating at 200 kV accelerating voltage. ICP-AES (Atomscan Advantage, Thermo Jarrell Ash, USA) was used to determine the concentration of metal species. NMR spectra were recorded on a Brucker-400 MHz spectrometer. The C and O K-edge X-ray absorption spectra were measured at beamline B12b of National Synchrotron Radiation Laboratory (NSRL, China) in the total electron yield (TEY) mode by collecting the sample drain current under a vacuum better than 1 × 10 –7 Pa.